Higher levels of sex chromosome heteromorphism are associated with markedly stronger reproductive isolation The two ‘rules of speciation’, Haldane’s rule and the large X-effect, describe the genetic basis of postzygotic isolation, and have led to the realization that sex chromosomes play an important role in this process. However, a range of sex determination mechanisms exists in nature, not always involving sex chromosomes. Based on these ‘rules of speciation’, I test the hypothesis that the presence of sex chromosomes will contribute to a faster evolution of intrinsic postzygotic isolation. I show that taxa that do not have sex chromosomes evolve lower levels of postzygotic isolation than taxa with sex chromosomes, at a similar amount of genetic divergence. Taxa with young homomorphic sex chromosomes show an intermediate pattern compared to taxa with heteromorphic sex chromosomes and taxa without sex chromosomes. These results are consistent with predictions from the two ‘rules of speciation’, and emphasize the importance of sex chromosomes for the evolution of intrinsic postzygotic isolation. The evolution of postzygotic reproductive isolation, by the formation of maladaptive hybrids, can often be explained by the accumulation of Dobzhansky–Muller incompatibilities (DMIs) between incipient species [1] , [2] . DMIs arise when alleles that are neutral or beneficial on the parental genetic background lead to deleterious effects in a hybrid background. Two ‘rules of speciation’ have been proposed to further describe patterns of the genetic basis of postzygotic isolation [3] . First, Haldane’s rule [4] states that whenever a sex is absent, rare or sterile in a cross between two taxa, that sex is usually the heterogametic sex. This rule is obeyed by a wide range of animal taxa and at least one group of plants that possess sex chromosomes [5] . The second rule is named the large X-effect, and is based on observation that the X (or Z) chromosome has a disproportionately high impact on hybrid fitness compared to autosomes. This has been shown, in Drosophila , to be due to a higher density of male sterility factors in the X chromosome [6] , [7] . Both ‘rules of speciation’ indicate that sex chromosomes are important in the formation of intrinsic postzygotic isolation (IPI) [8] . However, a variety of sex determination mechanisms exist in nature, ranging from heteromorphic sex chromosomes, where one of the chromosomes is largely degenerate, to the absence of sex chromosomes, where sex is determined by the environment, and/or by a combination of genic factors that are not on the same chromosome [9] . The transition between an absence of sex chromosomes and heteromorphic sex chromosomes is observed in taxa bearing ‘young’ sex chromosomes. Young sex chromosomes are usually homomorphic, where size and gene content are similar between the two chromosomes. As these chromosomes ‘age’, recombination decreases and the Y (W) chromosome starts to degenerate [9] . Considering the importance of sex chromosomes in the evolution of IPI, it has been proposed that speciation and IPI should evolve more slowly in taxa lacking sex chromosomes [10] , [11] , [12] , but no empirical evidence exists showing that the amount of IPI suffered by taxa bearing heteromorphic sex chromosomes is higher than that suffered by taxa without sex chromosomes. I therefore propose the following hypothesis: for a given amount of genetic divergence, higher sex chromosome heteromorphism will be accompanied by an increase in IPI. If taxa are classified based on their sex determination mechanism (as heteromorphic, homomorphic and no sex chromosomes), one would expect crosses between taxa in the heteromorphic sex chromosome group to display higher levels of IPI compared to the other two sex determination groups, and the homomorphic sex chromosome group should be intermediate. The homomorphic sex chromosome group spans a wide range of the sex chromosome evolution spectrum, so that taxa closer to the heteromorphic end of the spectrum should behave more like the heteromorphic sex chromosome group, while taxa on the opposite end of the spectrum should behave more like taxa without sex chromosomes. Three theories that explain Haldane’s rule and the large X-effect can further clarify the pattern proposed in the hypothesis. First, the dominance theory stems from the idea that DMIs are on average partially recessive [13] , [14] , [15] , in a way that the average effect of an incompatibility when heterozygous is less than half of the effect of that incompatibility when hemizygous. Incompatibilities will be partially masked in F 1 hybrids, since they are heterozygous, except when they are X-linked (in taxa with sex chromosomes), in which case they will be fully expressed in the hemizygous sex, leading to Haldane’s rule (but not the large X-effect). The amount of hemizygosity is relative to the amount of degeneracy between the sex chromosomes, so the dominance theory alone could lead to the pattern proposed above. Note that in this case the homogametic sex should suffer much lower levels of isolation in taxa where both copies of the X chromosome are active, such as Drosophila . In taxa where X inactivation occurs (such as in mammals), the strength of isolation may be higher in the homogametic sex as well, compared to taxa without sex chromosomes, especially in marsupials where only the paternal X is silenced [16] . Second, the faster X (Z) theory [17] predicts that genetic changes accumulate faster on the X chromosome than on autosomes, which occurs either because of efficient selection on hemizygous mutations when they are partially recessive [17] , or due to differences in effective population size between the X chromosome and autosomes [18] , both of which are dependent on the amount of degeneracy between the sex chromosomes. This process could lead to the faster accumulation of hybrid incompatibilities on the X chromosome the more differentiated the sex chromosomes are, and both Haldane’s rule and the large X-effect would be observed. Third, the faster-heterogametic-sex theory [19] explains the appearance of sterility in the heterogametic sex due to genomic conflicts, such as meiotic drive. If genomic conflicts affect sex ratio, there will be strong selection for suppressors to evolve. This evolutionary arms race will be stronger in the heterogametic sex, causing faster evolution of gametogenesis genes, and hence hybrid incompatibilities, leading to both Haldane’s rule and the large X-effect. The rate of this process is again dependent on the amount of degeneracy between sex chromosomes. Here I separate the large X-effect from the effects of dominance, where a large X-effect is caused by a higher density of incompatibilities accumulating on the X (Z) chromosome [6] , [7] , and not due to the fact that hemizygosity exposes incompatibilities in this chromosome (dominance theory). Of course, if the incompatibilities that stem from both faster X and/or faster-heterogametic-sex (which lead to the large X-effect) are on average partially recessive, we would observe an exaggerated pattern due to the combination of the large X-effect and the dominance theory [20] . In this study I show that taxa bearing heteromorphic sex chromosomes suffer higher levels of IPI than taxa with homomorphic and without sex chromosome. Taxa with homomorphic sex chromosomes display an intermediate pattern compared to the other sex chromosome groups. The cause of this is likely a combination of the dominance theory and the large X-effect, and emphasizes the importance of sex chromosomes for the evolution of postzygotic reproductive isolation. 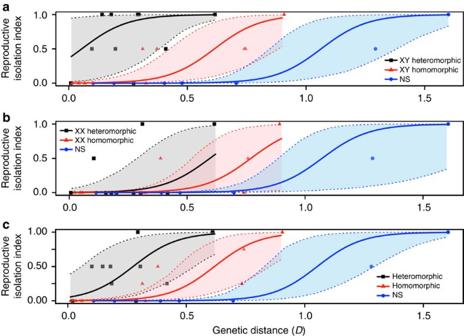Figure 1: Strength of total intrinsic postzygotic isolation versus Nei’sDgenetic distance. Regression lines were calculated through a logistic normal model. Logit values were transformed back to the reproductive isolation index values (from 0 to 1) for the purpose of visualization. Het=heteromorphic sex chromosomes (n=10); Hom=homomorphic sex chromosomes (n=9); NS=no sex chromosomes (n=7). (a) F1hybrids of the XY sex. (b) F1hybrids of the XX sex. (c) Both sexes analysed together. (a,c) Taxa with heteromorphic sex chromosomes suffer higher levels of intrinsic postzygotic isolation at lower genetic distances compared to the other two groups (t-test, FDR adjustedP=0.0252 for Het versus Hom,n=19; FDR adjustedP=0.0009 for Het versus NS,n=17). Species without sex chromosomes remain compatible until much higher levels of genetic differentiation (t-test, Hom versus NS:P=0.0346; FDR adjustedP=0.0967,n=16). (b) The heteromorphic sex chromosome group is significantly higher than the no sex chromosome group (t-test,P=0.0457,n=17), but the difference is not significant if corrections for multiple comparisons are carried out (FDR adjustedP=0.1028), while all other comparisons are not significantly different. All comparisons arepost-hocpairwiset-tests with 22 degrees of freedom. Colored bands are 95% bootstrap confidence intervals. Total intrinsic postzygotic isolation To test the proposed hypothesis, data on F 1 hybrid IPI were surveyed form the literature, for crosses between taxa with heteromorphic sex chromosomes, homomorphic sex chromosomes and taxa without sex chromosomes ( Table 1 and Supplementary Table 1 ). Postzygotic isolation was measured as in Coyne and Orr [21] , with values that go from 0 to 1, with a slight modification when sexes were analysed separately (Methods). I analysed the data in four different ways: heterogametic and homogametic sexes were analysed separately for total postzygotic isolation, and for inviability alone, and both sexes were analysed together for the same two measures of reproductive isolation. Table 1 Crosses data. Full size table I first analysed the data separating the heterogametic and homogametic sexes. To avoid confusion between the words hetero-/homogametic and hetero-/homomorphic, I refer to the heterogametic and homogametic sexes as XY and XX, respectively. For this analysis the IPI index was adapted to have three different values (0, 0.5, 1.0), where a score of 0 indicates that individuals of that sex are fertile and viable in both directions of the cross, a score of 0.5 indicates that sex is sterile or inviable in one direction of the cross, and a score of 1.0 indicates that sex is sterile or inviable in both directions of the cross. For the no sex chromosome group, which does not have XY and XX sexes, the scores are the same independent of which sex is analysed, since the cross with a score of 0.5 has unidirectional compatibility (both males and females are inviable in one direction of the cross, but viable and fertile in the other). For the XY sex data set the heteromorphic sex chromosome group reached higher levels of postzygotic isolation at lower genetic divergence than the homomorphic sex chromosome group ( t -test, P =0.0042, FDR adjusted P =0.0252, n= 19) and the no sex chromosome group ( t -test, P =0.0001, FDR adjusted P =0.0009, n= 17). 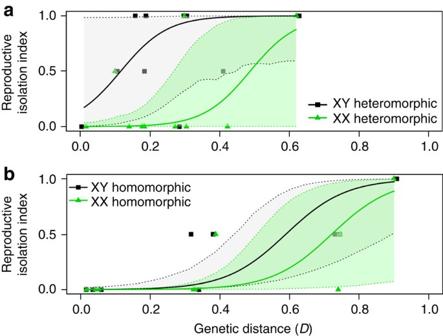Figure 2: Strength of intrinsic postzygotic isolation versus Nei’sDgenetic distance for XY and XX sexes in heteromorphic and homomorphic chromosome taxa. Regression lines were calculated through a logistic normal model. Logit values were transformed back to the reproductive isolation index values (from 0 to 1) for the purpose of visualization. (a) Crosses between taxa with heteromorphic sex chromosomes. The XY sex reaches higher levels of intrinsic postzygotic isolation at lower genetic distances than the XX sex (difference between intercepts=5.53;t-test,t(17)=2.32;P=0.0331,n=20). (b) Crosses between taxa with homomorphic sex chromosomes. Intrinsic postzygotic isolation is not significantly different between the two sexes (difference between intercepts=1.53;t-test,t(15)=1.02;P=0.3218,n=18). Colored bands are 95% bootstrap confidence intervals. The homomorphic sex chromosome group was intermediate and different from the other two groups (homomorphic versus no sex chromosome groups: t -test, P =0.0346, but the difference is not significant when multiple comparisons are accounted for: FDR adjusted P =0.0967, n= 16; Table 2 and Fig. 1a ). Table 2 Results from the linear model with the response variable (total IPI) logit transformed. Full size table Figure 1: Strength of total intrinsic postzygotic isolation versus Nei’s D genetic distance. Regression lines were calculated through a logistic normal model. Logit values were transformed back to the reproductive isolation index values (from 0 to 1) for the purpose of visualization. Het=heteromorphic sex chromosomes ( n =10); Hom=homomorphic sex chromosomes ( n =9); NS=no sex chromosomes ( n =7). ( a ) F 1 hybrids of the XY sex. ( b ) F 1 hybrids of the XX sex. ( c ) Both sexes analysed together. ( a , c ) Taxa with heteromorphic sex chromosomes suffer higher levels of intrinsic postzygotic isolation at lower genetic distances compared to the other two groups ( t -test, FDR adjusted P =0.0252 for Het versus Hom, n =19; FDR adjusted P =0.0009 for Het versus NS, n =17). Species without sex chromosomes remain compatible until much higher levels of genetic differentiation ( t -test, Hom versus NS: P =0.0346; FDR adjusted P =0.0967, n =16). ( b ) The heteromorphic sex chromosome group is significantly higher than the no sex chromosome group ( t -test, P =0.0457, n= 17), but the difference is not significant if corrections for multiple comparisons are carried out (FDR adjusted P =0.1028), while all other comparisons are not significantly different. All comparisons are post-hoc pairwise t -tests with 22 degrees of freedom. Colored bands are 95% bootstrap confidence intervals. Full size image When considering only the XX sex, however, the same pattern is not expected. If we assume incompatibilities appear at the same rate in both autosomes and sex chromosomes, and they are on average partially recessive (dominance theory, without any effect of sex chromosomes), crosses from all three sex chromosome groups should show similar amounts of postzygotic isolation for a given amount of genetic divergence since all individuals are heterozygous throughout their entire genome. Two conditions would lead to higher levels of isolation in the XX sex of taxa with sex chromosomes in this case: in a faster X scenario changes would accumulate faster on the X chromosome versus autosomes, which could increase the total number of incompatibilities (including X-X incompatibilities), and in some cases where dosage compensation inactivates one of the X chromosomes (as in mammals) making it effectively hemizygous. In this case however, the effect will not be as strong as in the heterogametic sex because there will be a mosaic pattern of inactivation of either of the X chromosomes across cells. In the XX sex data set, the heteromorphic and homomorphic sex chromosome groups were not significantly different from each other; nor was the homomorphic and no sex chromosome groups. The heteromorphic sex chromosome group did however experience a higher level of IPI than the no sex chromosome group ( t -test, P =0.0457, n= 17), but this difference was not significant when multiple comparisons were accounted for (FDR adjusted P =0.1028; Table 2 and Fig. 1b ). The main hypothesis, however, states that higher sex chromosome heteromorphism will be accompanied by an increase in IPI, and this should hold if the effects on both sexes are combined. When the sexes are analysed together, the resulting pattern is somewhat intermediate to the one we see when the sexes are analysed separately, and all groups are different from each other (the difference between homomorphic and heteromorphic sex chromosome groups, however, is marginally insignificant when FDR adjusted, P =0.0706; Table 2 ; Fig. 1c ). Haldane’s rule and unidirectional incompatibility A comparison between the XY and XX sex data sets within each sex determination group shows that the difference between the two sexes is higher for the heteromorphic sex chromosome group (the difference between the intercepts of both sexes is 5.53 for the logit transformed data, where the XY sex is significantly higher, t -test, P =0.0331, n= 20) than for the homomorphic sex chromosome group (1.53 intercept difference, and the two sexes are not significantly different, t -test, P =0.3218, n= 18; Fig. 2 ); as stated before, there is no difference between the sexes for the no sex chromosome group. These results show that Haldane’s rule evolves more readily with higher sex chromosome heteromorphism, while unidirectional incompatibility becomes more common with lower sex chromosome differentiation. Figure 2: Strength of intrinsic postzygotic isolation versus Nei’s D genetic distance for XY and XX sexes in heteromorphic and homomorphic chromosome taxa. Regression lines were calculated through a logistic normal model. Logit values were transformed back to the reproductive isolation index values (from 0 to 1) for the purpose of visualization. ( a ) Crosses between taxa with heteromorphic sex chromosomes. The XY sex reaches higher levels of intrinsic postzygotic isolation at lower genetic distances than the XX sex (difference between intercepts=5.53; t -test, t (17)=2.32; P =0.0331, n= 20). ( b ) Crosses between taxa with homomorphic sex chromosomes. Intrinsic postzygotic isolation is not significantly different between the two sexes (difference between intercepts=1.53; t -test, t (15)=1.02; P =0.3218, n= 18). Colored bands are 95% bootstrap confidence intervals. Full size image Intrinsic postzygotic isolation due to inviability Total IPI can be caused by both sterility and inviability, and there is evidence that sterility evolves more quickly than inviability [22] . Also, while evidence supports the dominance theory as an explanation of Haldane’s rule for both inviability and sterility, evidence for the large X-effect is restricted to cases of sterility [7] , [8] . I therefore analysed the data considering only viability ( Table 1 and Supplementary Table 1 ), as we would expect the difference between the sex chromosome groups to be smaller if the pattern observed in Fig. 1 is being driven by a combination of the dominance theory and the large X-effect. Note that since we cannot observe if inviable individuals are also sterile, the same analysis cannot be performed for sterility only. 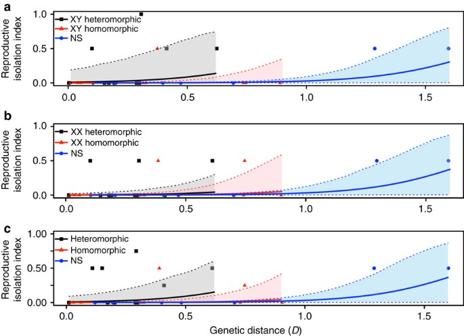Figure 3: Strength of intrinsic postzygotic isolation versus Nei’sDgenetic distance considering only viability. Regression lines were calculated through a logistic normal model. Logit values were transformed back to the reproductive isolation index values (from 0 to 1) for the purpose of visualization. Het=heteromorphic sex chromosomes (n=10); Hom=homomorphic sex chromosomes (n=9); NS=no sex chromosomes (n=7). (a) F1hybrids of the XY sex; (b) F1hybrids of the XX sex. (c) Both sexes analysed together. None of the comparisons are significantly different, except for the comparison of Het versus NS in (c), when both sexes are analysed together, where Het reaches higher levels of postzygotic isolation at lower genetic distance than NS (t-test,P=0.0376,n=17), although this difference is not significant when multiple comparisons are accounted for (FDR adjustedP=0.0967). All pairwise comparisons arepost-hoc t-tests with 22 degrees of freedom. Colored bands are 95% bootstrap confidence intervals. When only viability was considered, in the XY data set, the regression lines for the homomorphic and no sex chromosome groups were estimated to be nearly identical, while the difference between the heteromorphic sex group and the other two groups was larger but non significant ( Table 3 ; Fig. 3a ). In the XX data set there were no differences between the groups ( Fig. 3b ), and when both sexes were analysed together again the pattern was intermediate compared to when the sexes were analysed separately, and only the difference between the heteromorphic and no sex chromosome groups was significant ( t -test, P =0.0376 , n= 17), but not when multiple comparisons are accounted for (FDR adjusted P =0.0967; Table 3 ; Fig. 3c ). For the entire data set there are 20 cases where a sex is sterile, and 15 where a sex is inviable. The heteromorphic sex chromosome group has 10 sterile and 8 inviable sexes; the homomorphic sex chromosome group has 8 sterile and 3 inviable sexes; and the no sex chromosome group has 2 sterile and 4 inviable sexes ( Supplementary Table 1 ). Table 3 Results from the linear model with the response variable (IPI for viability only) logit transformed. Full size table Figure 3: Strength of intrinsic postzygotic isolation versus Nei’s D genetic distance considering only viability. Regression lines were calculated through a logistic normal model. Logit values were transformed back to the reproductive isolation index values (from 0 to 1) for the purpose of visualization. Het=heteromorphic sex chromosomes ( n =10); Hom=homomorphic sex chromosomes ( n =9); NS=no sex chromosomes ( n =7). ( a ) F 1 hybrids of the XY sex; ( b ) F 1 hybrids of the XX sex. ( c ) Both sexes analysed together. None of the comparisons are significantly different, except for the comparison of Het versus NS in ( c ), when both sexes are analysed together, where Het reaches higher levels of postzygotic isolation at lower genetic distance than NS ( t -test, P =0.0376, n= 17), although this difference is not significant when multiple comparisons are accounted for (FDR adjusted P =0.0967). All pairwise comparisons are post-hoc t -tests with 22 degrees of freedom. Colored bands are 95% bootstrap confidence intervals. Full size image In this study I showed that for a given amount of genetic divergence between two hybridizing species increasing sex chromosome heteromorphism is accompanied by a disproportionate increase in IPI ( Fig. 1 ). The effects of the dominance theory are clearly an important driver of this pattern, although these results suggest that the large X-effect also contributes to the observed pattern. Some support for this comes from a trend for higher levels of IPI suffered by the XX sex of the heteromorphic sex chromosome group compared to the no sex chromosome group (although this difference is not significant when multiple comparisons are accounted for ( Table 2 )). But more importantly, the presence of a large X-effect explains why inviability by itself does not separate the sex chromosome groups ( Fig. 3 and Table 3 ); this process appears to only lead to incompatibilities affecting sterility [6] , [7] . The present results also show that the prevalence of Haldane’s rule increases with increasing degeneracy of sex chromosomes, which means unidirectional incompatibility should become more common when the converse is true, as chromosomes between the two sexes are more similar ( Fig. 2 ). No single process is thought to cause Haldane’s rule by itself [23] , and this is also likely to be true for the large X-effect [8] . While evidence for the dominance theory is widespread [23] , cases supporting a large X-effect are less common at this point, but evidence exists in Anopheles [24] , Mus [25] and Drosophila [7] , [26] . The best evidence for a large X-effect comes from crosses between Drosophila mauritiana and D. sechellia [7] , where a higher density of incompatibilities causing hybrid male sterility were found to occur on the X chromosome than on autosomes, and these incompatibilities were found to be on average recessive. The mechanisms leading to a large X-effect are still debated, and both faster X (due to efficient selection of recessive mutations due to hemizygosity, or because of reduced effective population size of the hemizygous chromosome) and the faster-heterogametic-sex (due to genomic conflicts) could lead to a higher density of incompatibilities in the X chromosome. Evidence supporting a faster X as the cause of the large X-effect is contradictory in Drosophila depending on the cross and data set used, but is stronger in mammals, birds and moths (reviewed in Presgraves [8] and Meisel and Connallon [27] ). On the other hand, evidence that faster-heterogametic-sex (genomic conflict) can lead to the large X-effect is still rare, but two cases are known in Drosophila , where a correlation between genes that are involved in drive or suppression within species also lead to male hybrid sterility [28] , [29] , suggesting that these processes occur at least in some cases. Interestingly, the large X-effect only contributes to the evolution of sterility incompatibilities, which is evident in the results from Masly and Presgraves [7] , where the majority of incompatibilities that are X-linked contribute to sterility and not inviability. The same appears to be true for the results presented here, where inviability alone is not enough to explain the difference in total IPI between the different sex chromosome groups. Therefore, inviability may evolve at a similar rate in the different sex chromosome groups, and if they are not often X-linked their expression will also be more similar across the different sex chromosome groups. These results also appear to agree more with predictions from the faster-heterogametic-sex theory than with the faster X theory, since the former will lead only to sterility incompatibilities, while the latter, in theory, could lead to both sterility and inviability. Although given the current data set, where extremely divergent taxa are analysed together, this assertion should be taken with caution as different processes might be contributing to the evolution of DMIs in each group of taxa. The present study suggests that Haldane’s rule becomes prevalent with higher sex chromosome heteromorphism, while unidirectional incompatibilities are more important in taxa without sex chromosomes. This is consistent with what was observed in crosses between Drosophila species, where crosses between taxa with large X chromosomes obey Haldane’s rule at lower genetic distances than taxa with small X chromosomes [26] . Here this pattern is extended to the entire sex chromosome evolution spectrum, and it is observed that in taxa without sex chromosomes males and females are affected by DMI at similar rates. In this case, because incompatibilities are on average partially recessive, haploid uniparentally inherited factors may become especially important for the appearance of postzygotic barriers. If we consider the current results, where the IPI index depends on hybrids crossing a threshold (where one of the sexes is completely inviable or sterile) to reach a value of 0.25, there is no a priori reason to think that either sex would become inviable faster than the other in taxa without sex chromosomes. Similarly, hybrid sterility evolves at similar rates in both sexes in some taxa without sex chromosomes [30] , [31] despite the fact that sterility incompatibilities usually involve different loci for males and females [32] . If both sterility and inviability evolve at similar rates in both sexes, the IPI index will remain at 0, and will go to either 0.5 due to uniparentally inherited factors or 1 due to autosomal incompatibilities, mostly skipping the IPI index values of 0.25 and 0.75. This is precisely what is seen in Tigriopus californicus , where crosses between any two populations are fully compatible (IPI index of 0), unidirectionally compatible (IPI index of 0.5) or fully incompatible (IPI index of 1), in which case F 1 hybrids of both sexes are sterile in one direction and inviable in the other [33] , [34] . Such a pattern indicates that uniparentally inherited factors (likely cyto-nuclear incompatibilities in this case [35] ) may be of special importance for the formation of IPI in taxa without sex chromosomes. The different sex determination mechanisms form a continuum that goes from the complete absence of sex chromosomes to the presence of highly heteromorphic ones. This continuum is shown here to correlate with the level of IPI suffered between two taxa: increasing sex chromosome differentiation increases the severity of postzygotic isolation. Predictions from the two ‘rules of speciation’ are consistent with this pattern, and the current results accentuate the importance of sex chromosomes for the evolution of IPI, and highlight patterns that may be important in taxa that lack sex chromosomes. Crosses selection This survey included any crosses for which information was published for reciprocal crosses, sex determination mechanisms and Nei’s D genetic distances ( Table 1 and Supplementary Table 1 ). I used the same index of IPI as in Coyne and Orr [21] , where a score of 1 is assigned for every sex that is completely sterile or inviable in both reciprocal crosses. This sum is divided by 4, giving five possible scores: 0, 0.25, 0.50, 0.75 and 1. A score of 0 therefore indicates both males and females are viable and fertile in both directions of the cross, while a score of 1 indicates both males and females are either sterile or inviable. When analysing the XX and XY sexes separately, the IPI index was adapted to take three scores (0, 0.5 and 1), where a score of 0 indicates all individuals from this sex are fertile and viable in both directions of the cross, and a score of 1 indicates that sex is completely sterile or inviable in both directions of the cross. To avoid that the pattern in any of the sex chromosome groups was driven by a single taxon group, from all cases where information was available for more than three crosses (that is, Drosophila [21] , Lepidoptera [36] , frogs [37] and T. californicus [33] ), only three crosses with different IPI indexes were chosen. A large number of Drosophila crosses meet all the criteria outlined in the previous paragraph; however, some species of Drosophila have a neo-Y chromosome [38] ; therefore, I only included crosses for which I could confirm the Y chromosome was degenerate. For Lepidoptera, only 11 crosses from Presgraves [36] met all criteria, 7 of which had an isolation index of 0. Three crosses with different isolation indexes were randomly chosen in this case. In frogs, both male and female heterogamety exist, and the degree of sex chromosome differentiation as well as which sex is XY varies even in closely related species [39] . Of the crosses presented in Sasa et al. [37] , I included three crosses where information on sex chromosomes exists. Crosses from T. californicus were randomly chosen for three different isolation index values from Ganz and Burton [33] . Data that meet all the criteria are largely lacking for birds (mostly due to a lack of Nei’s D genetic distance for cases where reciprocal cross information exists), and only one cross was included. This is unfortunate since birds, in general, follow Haldane’s rule, but are known to evolve IPI much slower than other groups of animals [40] . The inclusion or omission of this single cross does not change the results presented here. In one cross, two types of sex determination mechanisms exist. Xiphophorus maculatus has a multi-factor sex determination mechanism (X, Y and W sex chromosomes), with male and female heterogamety, while X. helleri has polyfactorial sex determination, and neither sex is heterogametic [9] . The results are the same independent of assigning this cross to the no sex chromosome group or the homomorphic sex chromosome group. Genetic distance In order to compare the strength of isolation between these diverse groups of taxa, I only included taxa with published Nei’s D genetic distance [41] . This metric was chosen because it has been previously used in studies of this sort (i.e., refs 21 , 36 , 37 , 42 , 43 ) and it maximized the number of crosses in the analysis. Nei’s D measures the accumulation of codon differences at a locus between two taxa. Even if the molecular clocks are not the same between all the taxa analysed here, Nei’s D would still be a good metric as long as it approximates how divergent the genomes of the two hybridizing taxa are (Nei’s D is usually calculated based on information on at least 10 loci). If the genomes are not diverging at the same rate in distantly related taxa, we might expect DMIs to accumulate at different rates with respect to time as well. Here I am interested in finding how divergent the genomes are more so than time since divergence. Several other methods were attempted, such as calculating Ks , or four-fold degenerate transversions (4DTv) from DNA sequences. However, all of these methods yielded a very small number of potentially comparable crosses due to the lack of appropriate DNA sequences for many species, and in none of them was it possible to include the no sex chromosome group. Phylogenetic corrections Due to the small amount of data available, performing a traditional correction for phylogenetic dependence would render the data set too small for analysis. Therefore, the data set contains two groups of taxa with non-phylogenetic independent crosses ( Mus , and T. californicus ). To ameliorate this issue in these two groups the following criteria were applied: For Mus, the two crosses used are of increasing phylogenetic distance, which insures that the two crosses only shared a small portion of phylogenetic branch. Also, these crosses have different IPI indexes, meaning that even if a portion of the phylogenetic branch is not independent (certain incompatibilities may be part of both comparisons), we know that independent incompatibilities have evolved in each lineage since they last shared an ancestor leading to the difference in IPI. For T. californicus , the phylogenetic relationship of some of the populations is still unresolved; however, since this is the only group of crosses that yields IPI indexes greater than 0 in the no sex chromosome group, I decided to include three crosses that span the different IPI index classes observed in this group (0, 0.5, 1.0). Statistical analysis All statistical analyses were performed in R 2.15.1 (R Core Team 2012). Due to the nature of the IPI index, which is bounded by 0 and 1, analysis using an ordinary linear regression is inappropriate. However, when a logit transformation is applied to these values, this problem is eliminated. The IPI index values were logit transformed, and treated as a continuous variable. The logit function is undefined for values of 0 and 1, therefore I changed boundary values to 0.001 and 0.999 prior to logit transformation. Due to the small sample size in each sex chromosome group I used a logistic-normal model, which is an ordinary linear regression that uses the logit transformed IPI index as the response variable. This test is appropriate for small sample sizes because it uses an F -distribution (and a t -distribution for the post-hoc pairwise comparisons) with degrees of freedom that are a function of the sample size. An additive model was used, as there was not enough power to determine if the slopes were different (in an interactive model). This method was used in all comparisons presented in this study. In the present study, I am interested in the difference between the estimated regressions between each of the sex chromosome groups; therefore, the reported P -values in the results section refer to the post-hoc t -test for each pairwise comparison. To account for multiple comparisons a false discovery rate (FDR) [44] was used to adjust the P -values. Bootstrap confidence intervals Bootstrap confidence intervals for the predicted logit curves were obtained for each individual value of genetic distance using 1,000 bootstrap samples of the actual observations. This means that for each single combination of the predictors ‘genetic distance’ and ‘sex determination group’ we are 95% confident that the true inverse mean logit lies within the displayed interval for those specific predictor values. Influential observations Given the small number of observations in each sex chromosome group, I used standard diagnostic statistics to identify possible influential observations in the regression analysis. These were tests of leverage, Cook’s distance, DFFITS, and DFBETAS, all of which were run in R 2.15.1 (R Core Team 2012). The output of these tests is displayed in Supplementary Figs 1–4 and Supplementary Table 2 . None of the observations are influential given commonly used threshold values for these statistics. How to cite this article: Lima, T. G. Higher levels of sex chromosome heteromorphism are associated with markedly stronger reproductive isolation. Nat. Commun. 5:4743 doi: 10.1038/ncomms5743 (2014).